Alternative splicing ofCD44mRNA by ESRP1 enhances lung colonization of metastatic cancer cell In cancer metastasis, various environmental stressors attack the disseminating cells. The successful colonization of cancer cells in secondary sites therefore requires the ability of the cells to avoid the consequences of such exposure to the stressors. Here we show that orthotopic transplantation of a CD44 variant isoform-expressing (CD44v + ) subpopulation of 4T1 breast cancer cells, but not that of a CD44v − subpopulation, in mice results in efficient lung metastasis accompanied by expansion of stem-like cancer cells. Such metastasis is dependent on the activity of the cystine transporter xCT, and the stability of this protein is controlled by CD44v. We find that epithelial splicing regulatory protein 1 regulates the expression of CD44v, and knockdown of epithelial splicing regulatory protein 1 in CD44v + cells results in an isoform switch from CD44v to CD44 standard (CD44s), leading to reduced cell surface expression of xCT and suppression of lung colonization. The epithelial splicing regulatory protein 1-CD44v-xCT axis is thus a potential therapeutic target for the prevention of metastasis. Metastasis is the major cause of death for individuals with solid tumours [1] , largely because of the ineffectiveness of current therapies, once metastasis is established [2] , [3] . Metastasis is an inefficient process, however, with few cells released from a primary tumour eventually reinitiating tumour growth at distant sites. The formation of metastases has therefore been thought to result from the dissemination of stem-like cancer cells and their colonization of secondary sites [4] , [5] . The cell surface protein CD44 is a major marker for stem-like cancer cells [6] , [7] , [8] , [9] and is also highly expressed in metastatic cancer cells [4] , [6] . Although differences in CD44 + stem-like cells between primary tumours and metastases remain ill-defined, a subset of CD44 + stem-like cells in primary tumours might possess the ability to reinitiate tumour growth at distant sites [4] , [6] . It has remained largely unknown, however, whether CD44 is functionally associated with metastatic propagation by stem-like cancer cells. CD44 has been implicated in a variety of physiological processes in addition to cancer cell invasion and metastasis [10] , [11] , [12] , [13] . CD44 exists in numerous isoforms generated through alternative messenger RNA splicing [14] , with variability in the extracellular domain of CD44 being thought to underlie the functional diversity of this molecule [13] , [15] . A CD44 variant (CD44v) isoform containing v3 (the sequence encoded by variant exon 3) that undergoes heparin sulphate modification has thus been shown to interact with various growth factors including heparin-binding epidermal growth factor-like growth factor and basic fibroblast growth factor [16] , whereas the CD44v6 isoform has been shown to act as a co-receptor for the receptor tyrosine kinase c-Met [17] . Furthermore, we recently showed that interaction of CD44v8-10 with the cystine transporter xCT (SLC7A11) stabilizes the latter protein and thereby potentiates the ability of cancer cells to defend themselves against reactive oxygen species (ROS) [18] . The generation of CD44v isoforms might therefore modulate the activity of various plasma membrane proteins including receptor tyrosine kinases and transporters in cancer cells. Given that cancer cells are exposed to environmental stressors such as oxygen or nutrient deficiency, low pH, inflammatory mediators, and ROS during metastasis, the ability to avoid the consequences of such exposure is required for successful colonization by cancer cells [19] , [20] , [21] . The cystine transporter xCT functions as a Na + -independent transporter that mediates the exchange of extracellular cystine for intracellular glutamate and thereby promotes the synthesis of reduced glutathione (GSH) [22] , [23] , a ubiquitous reducing thiol peptide that serves as an important intracellular redox buffer and is associated with resistance of cancer cells to anticancer agents [24] , [25] . The availability of cysteine is rate-limiting for GSH synthesis [26] , and the activity of xCT is therefore essential for such resistance to anticancer agents [23] , [27] . However, the functional relevance of CD44v and xCT in the metastatic spread of stem-like cancer cells has remained undetermined. Here we show that CD44v–xCT expression regulated by ESRP1 in metastatic breast cancer cells confers the ability of evasion from oxidative stress and thereby promotes the lung metastasis. These findings suggest that CD44v may be a therapeutic target. Metastatic subpopulation in 4T1 cells expresses CD44v To investigate the role of CD44v in cancer metastasis, we studied the mouse breast cancer cell line 4T1 and its isogenic sublines (4T07, 168FARN, 67NR). All of these cells form primary tumours in mice, but only 4T1 cells give rise to visible lung metastases [28] ( Fig. 1a ). RT–PCR analysis revealed that the abundance of CD44v messenger RNA was markedly greater than that of CD44s mRNA in 4T1 cells, whereas only CD44s mRNA was detected in the nonmetastatic sublines ( Fig. 1b ; Supplementary Fig. S1 ). Flow cytometry showed that 4T1 cells consist of two subpopulations, CD44v + cells (which predominantly express CD44v) and CD44v − cells (which express only CD44s), whereas the nonmetastatic sublines consist only of CD44v − cells ( Fig. 1c ), suggesting that CD44v might be associated with the metastatic ability of 4T1 cells. We isolated the CD44v + and CD44v − subpopulations of 4T1 cells by fluorescence-activated cell sorting (FACS) and subjected these cells to immunoblot analysis and to analysis followed by direct sequencing of the PCR products [29] ( Supplementary Fig. S1 and Supplementary Methods ). The predominant CD44v isoform in the CD44v + cells was found to be CD44v8-10. Each subpopulation was transplanted (1×10 5 cells) into mouse mammary glands. The incidence (CD44v + , 13/13; CD44v − , 11/11) and volume ( Fig. 1d ) of the primary tumours derived from CD44v + or CD44v − cells were similar. However, the incidence of lung metastasis by CD44v + cells was markedly higher than that of CD44v − cells (CD44v + , 13/13; CD44v − , 3/11), and both IntegriSense quantitative fluorescence imaging [30] and histological analysis revealed that the extent of lung metastatic lesions derived from CD44v + cells was greater than that of those formed by CD44v − cells ( Fig. 1e,f ). The CD44v + subpopulation was thus enriched in highly metastatic cells compared with the CD44v − subpopulation. 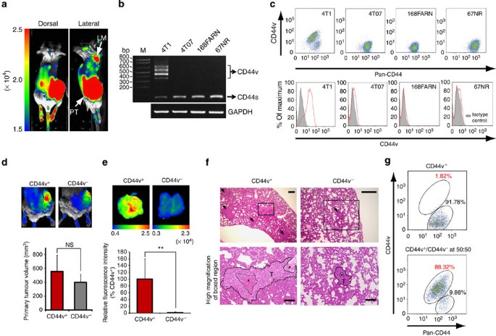Figure 1: Expression of CD44v in metastatic breast cancer cells with lung colonization potential. (a) IntegriSense fluorescence images of a representative mouse injected with 4T1 cells (1×105) orthotopically into the mammary gland. Left colour bar and associated numbers indicate fluorescence intensity levels, with red and blue representing high and low fluorescence signals, respectively. LM, lung metastasis; PT, primary tumour. (b) RT–PCR analysis of total RNA from the indicated cell lines with primers targeted to exons 5 and 16 of the mouseCD44gene as well as to the mouseglyceraldehyde-3-phosphate dehydrogenase(Gapdh) gene (internal control). M, DNA size marker. (c) Flow cytometric analysis of CD44 isoform expression on the indicated cell lines with antibodies that recognize all isoforms of CD44 (pan-CD44) or only CD44v. Similar results were obtained in three independent experiments. (d) IntegriSense images of primary tumours formed as a result of orthotopic injection of sorted CD44v+or CD44v−4T1 cells (1×105) into the mammary gland of mice (upper). Tumour volume at 30 days after cell injection was calculated as length×(width)2/2 (bottom), and data are means±s.d. for eight animals per group. NS, not significant. (e) IntegriSense images of lung metastases formed in mice injected as in (d), and quantitative analysis of the total fluorescence intensity per lung metastatic lesion. Quantitative data are means±s.d. for 5 animals injected with CD44v+cells or CD44v−cells. **P<0.01 (Student'st-test). (f) Haematoxylin-eosin staining of lung metastases formed 30 days after orthotopic injection of CD44v+or CD44v−cells into the mammary gland of recipient mice. The boxed regions in the upper panels are shown at higher magnification in the lower panels. Arrows indicate metastatic nodules in the lung; asterisks indicate blood vessels; T, tumour. Scale bars, 300 μm (upper) or 100 μm (lower). (g) Flow cytometric analysis of CD44 isoform expression on tumour cells (6-TG-resistant and lineage marker-negative (Lin−) cells) isolated from lung metastases at 30 days after intravenous injection of CD44v−4T1 cells (1×104) or both CD44v+and CD44v−4T1 cells (5×103cells each). Figure 1: Expression of CD44v in metastatic breast cancer cells with lung colonization potential. ( a ) IntegriSense fluorescence images of a representative mouse injected with 4T1 cells (1×10 5 ) orthotopically into the mammary gland. Left colour bar and associated numbers indicate fluorescence intensity levels, with red and blue representing high and low fluorescence signals, respectively. LM, lung metastasis; PT, primary tumour. ( b ) RT–PCR analysis of total RNA from the indicated cell lines with primers targeted to exons 5 and 16 of the mouse CD44 gene as well as to the mouse glyceraldehyde-3-phosphate dehydrogenase ( Gapdh ) gene (internal control). M, DNA size marker. ( c ) Flow cytometric analysis of CD44 isoform expression on the indicated cell lines with antibodies that recognize all isoforms of CD44 (pan-CD44) or only CD44v. Similar results were obtained in three independent experiments. ( d ) IntegriSense images of primary tumours formed as a result of orthotopic injection of sorted CD44v + or CD44v − 4T1 cells (1×10 5 ) into the mammary gland of mice (upper). Tumour volume at 30 days after cell injection was calculated as length×(width) 2 /2 (bottom), and data are means±s.d. for eight animals per group. NS, not significant. ( e ) IntegriSense images of lung metastases formed in mice injected as in ( d ), and quantitative analysis of the total fluorescence intensity per lung metastatic lesion. Quantitative data are means±s.d. for 5 animals injected with CD44v + cells or CD44v − cells. ** P <0.01 (Student's t -test). ( f ) Haematoxylin-eosin staining of lung metastases formed 30 days after orthotopic injection of CD44v + or CD44v − cells into the mammary gland of recipient mice. The boxed regions in the upper panels are shown at higher magnification in the lower panels. Arrows indicate metastatic nodules in the lung; asterisks indicate blood vessels; T, tumour. Scale bars, 300 μm (upper) or 100 μm (lower). ( g ) Flow cytometric analysis of CD44 isoform expression on tumour cells (6-TG-resistant and lineage marker-negative (Lin − ) cells) isolated from lung metastases at 30 days after intravenous injection of CD44v − 4T1 cells (1×10 4 ) or both CD44v + and CD44v − 4T1 cells (5×10 3 cells each). Full size image Given that 4T1 cells are resistant to 6-thioguanine (6-TG) [28] , we isolated tumour cells by 6-TG selection from lung metastases formed after injection of CD44v − cells into the tail vein. Small metastatic nodules consisted mostly of CD44v − cells, suggesting that CD44v − cells also possess metastasis-initiating ability ( Fig. 1g ). However, when CD44v + and CD44v − cells were injected at a 50:50 ratio, lung metastases consisted mostly of CD44v + cells ( Fig. 1g ), indicating that the lung colonization potential of CD44v + cells is much higher than that of CD44v − cells. ESRP1 promotes lung metastasis of 4T1 cells To identify the mechanism underlying lung colonization potential, we performed microarray analysis ( Supplementary Methods ) followed by gene set enrichment analysis (GSEA) [31] . The CD44v + cell/CD44v − cell gene set profile was similar to the embryonic stem (ES) cell/mouse embryonic fibroblast (MEF) and induced pluripotent stem (iPS) cell/MEF profiles ( Fig. 2a ). CD44v + cells thus manifest an ES cell-like gene signature when compared with CD44v − cells. The gene for epithelial splicing regulatory protein 1 (ESRP1), which regulates alternative splicing of CD44 mRNA [14] , was highly expressed not only in CD44v + 4T1 cells but also in ES and iPS cells ( Supplementary Data 1 ). We therefore examined the role of this protein in metastasis. An ES cell-like gene expression signature has been associated with an aggressive phenotype in cancer [32] , and so we examined the relation between ESRP1 expression and prognosis with the use of gene expression profiles of breast cancer patients [33] . A high level of ESRP1 expression was significantly associated with a lower rate of overall survival ( Fig. 2b ), suggesting that increased ESRP1 expression is related to the malignant behaviour of human breast cancer. 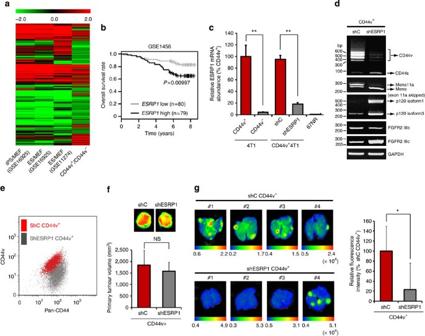Figure 2: Regulation of alternative splicing of CD44 mRNA and promotion of lung metastasis by ESRP1. (a) GSEA of microarray data for CD44v+cell/CD44v−cell, ES cell/MEF (GSE16925 and GSE11274), and iPS cell/MEF (GSE16925) profiles. (b) Kaplan–Meier plots of overall survival according toESRP1(219121_s_at) expression level for a breast cancer patient set (GSE1456,n=159). (c) Quantitative RT–PCR analysis of the abundance ofESRP1mRNA in CD44v−4T1 cells, shC CD44v+cells, shESRP1 CD44v+cells, and 67NR cells relative to that in CD44v+4T1 cells. Data were normalized by the amount ofGapdhmRNA and are means±s.d. from three independent experiments. **P<0.01 (Student'st-test). (d) RT–PCR analysis of splice variant mRNAs forCD44,Mena,p120 catenin,andFGFR2in shC CD44v+and shESRP1 CD44v+cells. (e) Flow cytometric analysis of CD44 expression on shC CD44v+and shESRP1 CD44v+cells with antibodies to pan-CD44 and to CD44v. (f) IntegriSense images of primary tumours formed in mice by orthotopically injected shC CD44v+or shESRP1 CD44v+cells (1×105) as well as tumour volume at 30 days after cell injection. Quantitative data are means±s.d. for five animals per group. (g) IntegriSense images of lung metastases and quantitative analysis of the total fluorescence signal intensity per lung metastatic lesion for mice injected as in (f). Quantitative data are means±s.d. for four animals per group. *P<0.05 (Student'st-test). Figure 2: Regulation of alternative splicing of CD44 mRNA and promotion of lung metastasis by ESRP1. ( a ) GSEA of microarray data for CD44v + cell/CD44v − cell, ES cell/MEF (GSE16925 and GSE11274), and iPS cell/MEF (GSE16925) profiles. ( b ) Kaplan–Meier plots of overall survival according to ESRP1 (219121_s_at) expression level for a breast cancer patient set (GSE1456, n =159). ( c ) Quantitative RT–PCR analysis of the abundance of ESRP1 mRNA in CD44v − 4T1 cells, shC CD44v + cells, shESRP1 CD44v + cells, and 67NR cells relative to that in CD44v + 4T1 cells. Data were normalized by the amount of Gapdh mRNA and are means±s.d. from three independent experiments. ** P <0.01 (Student's t -test). ( d ) RT–PCR analysis of splice variant mRNAs for CD44 , Mena , p120 catenin, and FGFR2 in shC CD44v + and shESRP1 CD44v + cells. ( e ) Flow cytometric analysis of CD44 expression on shC CD44v + and shESRP1 CD44v + cells with antibodies to pan-CD44 and to CD44v. ( f ) IntegriSense images of primary tumours formed in mice by orthotopically injected shC CD44v + or shESRP1 CD44v + cells (1×10 5 ) as well as tumour volume at 30 days after cell injection. Quantitative data are means±s.d. for five animals per group. ( g ) IntegriSense images of lung metastases and quantitative analysis of the total fluorescence signal intensity per lung metastatic lesion for mice injected as in ( f ). Quantitative data are means±s.d. for four animals per group. * P <0.05 (Student's t -test). Full size image The abundance of ESRP1 mRNA was significantly higher in CD44v + 4T1 cells than in CD44v − 4T1 cells and 67NR cells ( Fig. 2c ), suggesting that ESRP1 regulates CD44v expression. We established CD44v + 4T1 cells that stably express either a short hairpin RNA (shRNA) specific for ESRP1 mRNA (shESRP1 CD44v + cells) or a corresponding scrambled (control) shRNA (shC CD44v + cells) ( Supplementary Methods ). ESRP1 knockdown resulted in a switch in CD44 mRNA splicing that led to the generation of the CD44 standard isoform (CD44s) mRNA rather than CD44v mRNA ( Fig. 2d ). Furthermore, the mRNAs for Mena, fibroblast growth factor receptor 2 (FGFR2), and p120 catenin, whose splicing is also regulated by ESRP1 (ref. 14 ), underwent a shift in splicing pattern in shESRP1 CD44v + cells ( Fig. 2d ). Flow cytometry also revealed that ESRP1 depletion resulted in a pronounced conversion from the production of CD44v to that of CD44s without an effect on the overall level of CD44 expression ( Fig. 2e ). To determine whether ESRP1 contributes to the metastatic behaviour of CD44v + cells, we transplanted shC CD44v + or shESRP1 CD44v + cells orthotopically into mouse mammary glands. Although the incidence (shC CD44v + , 15/15; shESRP1 CD44v + , 15/15) and volume ( Fig. 2f ) of primary tumours formed by these cells were similar, the incidence of lung metastasis was reduced for the ESRP1-depleted cells (shC CD44v + , 14/15; shESRP1 CD44v + , 6/15). Furthermore, the extent of lung metastases was reduced for shESRP1 CD44v + cells compared with shC CD44v + cells ( Fig. 2g ), suggesting that ESRP1 promotes lung colonization by CD44v + 4T1 cells. CD44v + stem-like cells dominantly colonize and expand in the lung We next examined whether metastasis-associated stress results in enrichment of ROS-resistant cells. We isolated tumour cells from the primary lesion (4T1PT) and lung metastases (4T1LM) formed by 4T1 cells ( Fig. 3a ) and evaluated their intracellular ROS levels by staining with the fluorescent probe 2′,7′-dichlorofluorescein diacetate (DCFH-DA). ROS levels of 4T1LM cells were lower than those of 4T1PT cells in the absence or presence of hydrogen peroxide (H 2 O 2 ) ( Fig. 3b ; Supplementary Fig. S2 ), indicating that 4T1LM cells have a higher ROS-defence capacity than 4T1PT cells. Furthermore, flow cytometry of cells labelled with 5-chloromethylfluorescein diacetate (CFMDA), a fluorescent probe for GSH ( Supplementary Methods ), revealed that intracellular GSH abundance in 4T1LM cells was greater than that of 4T1 or 4T1PT cells ( Fig. 3c ). A luminescence-based assay that relies on the conversion of a luciferin derivative to luciferin in the presence of GSH [18] also showed that the intracellular GSH content of 4T1LM cells was significantly greater than that of 4T1PT cells ( Supplementary Fig. S2 ). Together, these results indicated that lung metastasis results in enrichment of ROS-resistant cells with high GSH levels. To examine whether CD44v-expressing cells maintain high GSH levels in vivo , we applied imaging mass spectrometry to visualize GSH and oxidized glutathione (GSSG) in frozen tissue samples [34] , [35] . CD44v + lung metastases formed by 4T1 cells manifested high levels of GSH but not of GSSG ( Fig. 3d ), suggesting that CD44v confers ROS resistance to cancer cells through the promotion of GSH synthesis. We then examined the role of GSH in lung colonization by CD44v + cells with the use of L -buthionine sulphoximine (BSO), which inhibits γ-glutamylcysteine synthase [36] and thereby depletes intracellular GSH ( Supplementary Fig. S2 ). Lung colonization by L -buthionine sulphoximine-treated CD44v + cells was significantly inhibited compared with that of control cells ( Supplementary Fig. S2 ), suggesting that a high intracellular GSH level enhances the lung colonization potential of CD44v + cells. 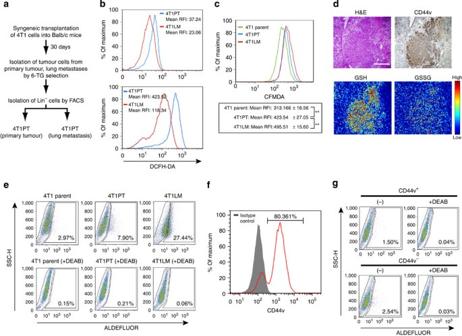Figure 3: Selective expansion of CD44v+stem-like cancer cells during lung metastasis. (a) Experimental protocol. (b) 4T1PT or 4T1LM cells were incubated with or without 500 μM H2O2for 20 min, stained with DCFH-DA, and subjected to flow cytometric analysis. RFI, relative fluorescence intensity. Similar results were obtained in three independent experiments. (c) Flow cytometric analysis of parental 4T1 as well as 4T1PT and 4T1LM cells stained with CFMDA (upper). Mean±s.d. values for RFI from five independent experiments are also shown (lower); **P<0.01(Student'st-test). (d) Haematoxylin-eosin (H&E) staining and immunohistochemical staining of CD44v (upper panels) as well as imaging mass spectrometry of GSH and GSSG (lower panels) in lung metastases formed by 4T1 cells. The colour bar indicates peak intensity levels atm/z306.0 (GSH) or 611.1 (GSSG), with red and blue representing high and low signals, respectively. Scale bar, 500 μm. (e) Flow cytometry of 4T1, 4T1PT, or 4T1LM cells incubated with the ALDEFLUOR substrate (BAAA) with or without the specific inhibitor (DEAB) to establish the baseline fluorescence and to define the ALDEFLUOR-positive region. SSC-H, side scatter. (f) Flow cytometric analysis of CD44v expression in ALDEFLUOR-positive 4T1LM cells. Cells were stained with antibodies to CD44v after incubation with BAAA in the absence or presence of DEAB. Similar results were obtained in three independent experiments. (g) Flow cytometric analysis of CD44v+or CD44v−4T1 cells subjected to the ALDEFLUOR assay as in (e). Similar results were obtained in three independent experiments. Figure 3: Selective expansion of CD44v + stem-like cancer cells during lung metastasis. ( a ) Experimental protocol. ( b ) 4T1PT or 4T1LM cells were incubated with or without 500 μM H 2 O 2 for 20 min, stained with DCFH-DA, and subjected to flow cytometric analysis. RFI, relative fluorescence intensity. Similar results were obtained in three independent experiments. ( c ) Flow cytometric analysis of parental 4T1 as well as 4T1PT and 4T1LM cells stained with CFMDA (upper). Mean±s.d. values for RFI from five independent experiments are also shown (lower); ** P <0.01(Student's t -test). ( d ) Haematoxylin-eosin (H&E) staining and immunohistochemical staining of CD44v (upper panels) as well as imaging mass spectrometry of GSH and GSSG (lower panels) in lung metastases formed by 4T1 cells. The colour bar indicates peak intensity levels at m/z 306.0 (GSH) or 611.1 (GSSG), with red and blue representing high and low signals, respectively. Scale bar, 500 μm. ( e ) Flow cytometry of 4T1, 4T1PT, or 4T1LM cells incubated with the ALDEFLUOR substrate (BAAA) with or without the specific inhibitor (DEAB) to establish the baseline fluorescence and to define the ALDEFLUOR-positive region. SSC-H, side scatter. ( f ) Flow cytometric analysis of CD44v expression in ALDEFLUOR-positive 4T1LM cells. Cells were stained with antibodies to CD44v after incubation with BAAA in the absence or presence of DEAB. Similar results were obtained in three independent experiments. ( g ) Flow cytometric analysis of CD44v + or CD44v − 4T1 cells subjected to the ALDEFLUOR assay as in ( e ). Similar results were obtained in three independent experiments. Full size image Breast cancer stem cells manifest an increased ROS defence capacity relative to their nontumorigenic progeny [37] . We therefore examined 4T1LM cells for the presence of stem-like cells with the use of ALDEFLUOR, a fluorescent probe for aldehyde dehydrogenase (ALDH) activity, a marker for stem-like cancer cells [38] . 4T1LM cells contained a much larger proportion of ALDEFLUOR-positive cells compared with 4T1 or 4T1PT cells ( Fig. 3e ). Furthermore, most ALDEFLUOR-positive 4T1LM cells expressed CD44v ( Fig. 3f ), suggesting that CD44v + stem-like cells may expand during lung colonization. In contrast, the proportions of ALDEFLUOR-positive cells among noninjected CD44v + or CD44v − 4T1 cells were similar ( Fig. 3g ). These results suggested that the difference in metastatic behaviour between CD44v + and CD44v − cells is determined by the difference in ROS resistance rather than by a difference in the size of the pre-existing stem-like cell population. CD44 splicing enhances ROS defence in metastatic 4T1 cells We examined the role of xCT in lung metastasis and found that the level of xCT expression on the surface of 4T1 cells was greater than that on 67NR (nonmetastatic) cells ( Fig. 4a ). It was also higher on CD44v + cells compared with CD44v − cells. xCT was downregulated on CD44v + cells by RNA interference-mediated depletion of ESRP1 ( Fig. 4b ), suggesting that ESRP1-dependent splicing of CD44 mRNA controls the cell surface expression of xCT. Consistent with these results ( Fig. 4a,b ), the intracellular GSH content was significantly higher for 4T1 cells than for 67NR cells, for CD44v + cells compared with CD44v − cells, and in shC CD44v + cells compared with shESRP1 CD44v + cells ( Fig. 4c ). These findings suggested that ESRP1-regulated CD44v expression increases the amount of xCT at the cell surface and thereby contributes to the maintenance of high GSH levels. To investigate whether xCT activity promotes lung colonization by CD44v-expressing cells, we examined the effect of the specific xCT inhibitor sulfasalazine ( Supplementary Methods ) [18] , [39] . Two weeks after intravenous injection of CD44v + cells, lung metastasis was suppressed in sulfasalazine-treated mice compared with saline-treated controls ( Fig. 4d ), suggesting that xCT has a functional role in lung colonization. 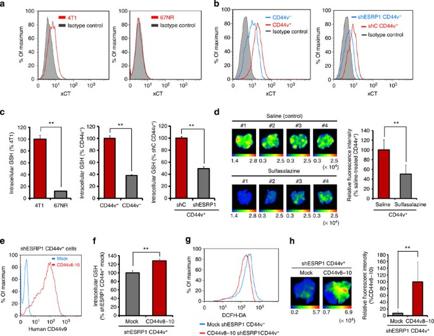Figure 4: CD44 splicing enhances ROS defence and lung colonization potential. (a) Flow cytometric analysis of xCT expression on 4T1 or 67NR cells. (b) Flow cytometry of xCT expression on CD44v+or CD44v−4T1 cells (upper left) and on shC CD44v+or shESRP1 CD44v+cells (upper right). CD44v−(Mean RFI; 6.72±0.14), CD44v+(Mean RFI; 10.06±0.93**). shESRP1 CD44v+(Mean RFI; 6.09±0.29), shC CD44v+(Mean RFI; 9.41±0.44**). Mean±s.d. values for RFI from five independent experiments. **P<0.01 (Student'st-test). (c) Intracellular GSH content of 4T1 or 67NR cells (left), CD44v+or CD44v−4T1 cells (middle), and shC CD44v+or shESRP1 CD44v+cells (right). Data are means±s.d. from five independent experiments. **P<0.01 (Student'st-test). (d) IntegriSense images of lung metastases formed in mice 2 weeks after intravenous injection of CD44v+cells (1×105) and the onset of treatment with sulfasalazine or saline. The fluorescence signal intensity of each lung metastasis was also measured; data are means±s.d. for four animals treated with saline and six animals treated with sulfasalazine. **P<0.01 (Student'st-test). (e) Flow cytometric analysis of human CD44v9 expression on the surface of shESRP1 CD44v+cells stably expressing human CD44v8-10 or stably transfected with the empty vector (mock). (f) Intracellular GSH content of cells transfected as in (e). Data are means±s.d. from five independent experiments. **P<0.01 (Student'st-test). (g) Mock-transfected or CD44v8-10-expressing shESRP1 CD44v+cells were incubated with 500 μM H2O2for 20 min, stained with DCFH-DA, and subjected to flow cytometric analysis. Mock-transfected shESRP1 CD44v+(Mean RFI; 232.73±4.89), CD44v8-10-expressing shC CD44v+(Mean RFI; 160.19±8.82**). Mean±s.d. values of RFI from five independent experiments. **P<0.01 (Student'st-test). (h) IntegriSense images of lung metastases formed 30 days after orthotopic injection of cells (1×105) transfected as in (e) into the mammary gland of recipient mice. The fluorescence signal intensity of each lung metastasis was also measured; data are means±s.d. for five animals per group. **P<0.01 (Student'st-test). Figure 4: CD44 splicing enhances ROS defence and lung colonization potential. ( a ) Flow cytometric analysis of xCT expression on 4T1 or 67NR cells. ( b ) Flow cytometry of xCT expression on CD44v + or CD44v − 4T1 cells (upper left) and on shC CD44v + or shESRP1 CD44v + cells (upper right). CD44v − (Mean RFI; 6.72±0.14), CD44v + (Mean RFI; 10.06±0.93**). shESRP1 CD44v + (Mean RFI; 6.09±0.29), shC CD44v + (Mean RFI; 9.41±0.44**). Mean±s.d. values for RFI from five independent experiments. ** P <0.01 (Student's t -test). ( c ) Intracellular GSH content of 4T1 or 67NR cells (left), CD44v + or CD44v − 4T1 cells (middle), and shC CD44v + or shESRP1 CD44v + cells (right). Data are means±s.d. from five independent experiments. ** P <0.01 (Student's t -test). ( d ) IntegriSense images of lung metastases formed in mice 2 weeks after intravenous injection of CD44v + cells (1×10 5 ) and the onset of treatment with sulfasalazine or saline. The fluorescence signal intensity of each lung metastasis was also measured; data are means±s.d. for four animals treated with saline and six animals treated with sulfasalazine. ** P <0.01 (Student's t -test). ( e ) Flow cytometric analysis of human CD44v9 expression on the surface of shESRP1 CD44v + cells stably expressing human CD44v8-10 or stably transfected with the empty vector (mock). ( f ) Intracellular GSH content of cells transfected as in ( e ). Data are means±s.d. from five independent experiments. ** P <0.01 (Student's t -test). ( g ) Mock-transfected or CD44v8-10-expressing shESRP1 CD44v + cells were incubated with 500 μM H 2 O 2 for 20 min, stained with DCFH-DA, and subjected to flow cytometric analysis. Mock-transfected shESRP1 CD44v + (Mean RFI; 232.73±4.89), CD44v8-10-expressing shC CD44v + (Mean RFI; 160.19±8.82**). Mean±s.d. values of RFI from five independent experiments. ** P <0.01 (Student's t -test). ( h ) IntegriSense images of lung metastases formed 30 days after orthotopic injection of cells (1×10 5 ) transfected as in ( e ) into the mammary gland of recipient mice. The fluorescence signal intensity of each lung metastasis was also measured; data are means±s.d. for five animals per group. ** P <0.01 (Student's t -test). Full size image ESRP1 affects the splicing of mRNAs for various proteins including FGFR2, p120 catenin, and Mena as well as CD44 (ref. 14 ). To examine the contribution of CD44v to ESRP1-dependent lung metastasis, we introduced CD44v8-10 complementary DNA [18] into shESRP1 CD44v + cells to generate cells that stably express CD44v8-10 as well as ESRP1 shRNA ( Fig. 4e ; Supplementary Fig. S3 ). Cells expressing CD44v8-10 showed a significantly higher level of GSH compared with cells transfected with the empty vector ( Fig. 4f ). Furthermore, the increase in ROS level after exposure to H 2 O 2 was reduced by forced expression of CD44v8-10 ( Fig. 4g ), indicating that CD44v8-10 expression enhanced ROS defence in ESRP1-depleted cells. ROS abundance in the absence of H 2 O 2 was not affected by CD44v8-10 expression ( Supplementary Fig. S3 ), suggesting that CD44v8-10 protects cancer cells on exposure to excessive amounts of ROS. Finally, forced expression of CD44v8-10 resulted in a marked increase in the lung metastatic potential of ESRP1-depleted cells ( Fig. 4h ). Together, these data suggested that alternative splicing of CD44 mRNA regulated by ESRP1 enhances xCT-dependent ROS defence in cancer cells and thereby promotes efficient lung colonization. Epigenetic regulation of ESRP1 expression in 4T1 cells ESRP1 expression was recently shown to be downregulated in cells undergoing the epithelial-mesenchymal transition (EMT) [40] . To investigate the relevance of EMT status to ESRP1 expression in CD44v + and CD44v − 4T1 cells, we examined the expression of EMT markers and Twist, an EMT-inducing transcription factor that is highly expressed in 4T1 cells [41] . Immunoblot analysis showed that both CD44v + and CD44v − cells express the epithelial markers E-cadherin and ZO-1 and that the expression level of Twist was similar in the two cell subpopulations ( Fig. 5a ), suggesting that ESRP1 expression in CD44v + and CD44v − 4T1 cells is regulated independently of EMT-related mechanisms. 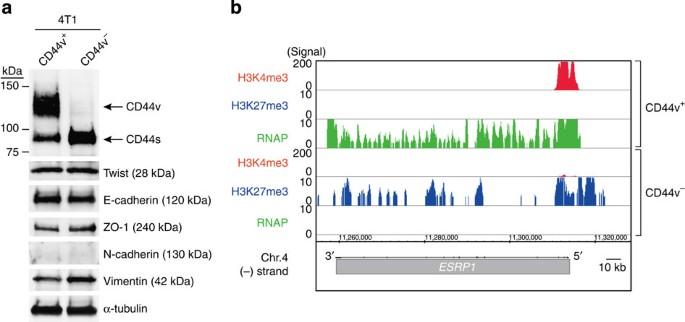Figure 5: EMT marker expression and epigenetic status of theESRP1locus in CD44v+or CD44v−4T1 cells. (a) Immunoblot analysis of the epithelial markers (E-cadherin and ZO-1) and the mesenchymal markers (N-cadherin and Vimentin) and Twist expression in CD44v+or CD44v−4T1 cells. α-Tubulin was analysed as a loading control. (b) Enrichment of histone H3K4me3 and H3K27me3 as well as of RNA polymerase II (RNAP) at theESRP1locus on mouse chromosome 4 in CD44+or CD44−4T1 cells as visualized with the 390-kbp UCSC mm9 genome browser. The gene is transcribed from right to left. Figure 5: EMT marker expression and epigenetic status of the ESRP1 locus in CD44v + or CD44v − 4T1 cells. ( a ) Immunoblot analysis of the epithelial markers (E-cadherin and ZO-1) and the mesenchymal markers (N-cadherin and Vimentin) and Twist expression in CD44v + or CD44v − 4T1 cells. α-Tubulin was analysed as a loading control. ( b ) Enrichment of histone H3K4me3 and H3K27me3 as well as of RNA polymerase II (RNAP) at the ESRP1 locus on mouse chromosome 4 in CD44 + or CD44 − 4T1 cells as visualized with the 390-kbp UCSC mm9 genome browser. The gene is transcribed from right to left. Full size image Posttranscriptional modifications of histones that affect chromatin structure influence ESRP1-mediated alternative splicing [42] , [43] , suggesting that alternative splicing is tightly regulated at the chromatin level. We therefore examined whether ESRP1 expression might also be regulated epigenetically through histone modification by performing chromatin immunoprecipitation (ChIP) sequencing analysis of the ESRP1 locus in CD44v + and CD44v − cells. CD44v + cells manifested a marked increase in the amount of trimethylated lysine-4 of histone H3 (H3K4me3), which marks open chromatin and active transcription [44] , compared with CD44v − cells ( Fig. 5b ). Conversely, the amount of trimethylated lysine-27 of histone H3 (H3K27me3), which is associated with gene silencing [45] , was increased in CD44v − cells ( Fig. 5b ). Consistent with these histone profiles, RNA polymerase II was enriched at the ESRP1 locus in CD44v + cells compared with CD44v − cells ( Fig. 5b ). Together, these findings suggested that ESRP1 expression in metastatic cancer cells is controlled at the chromatin level. Alternative splicing generates multiple mRNAs from a single-gene transcript, thereby greatly expanding proteomic diversity. Although only a small number of cell type-specific splicing regulators have been identified in mammals, numerous additional regulators will likely be found among the large number of uncharacterized RNA-binding proteins. ESRPs regulate the splicing of transcripts for epithelial- or mesenchymal-specific isoforms of proteins including CD44, FGFR2, p120 catenin, and Mena [14] . The expression of CD44v but not CD44s has been shown to promote the aggressive behaviour in several types of cancer cells including pancreatic cancer [10] , [46] and lymphoma [47] . We have now shown that depletion of ESRP1 in metastatic breast cancer cells changed the phenotype of these cells from CD44v + to CD44s + , without affecting the overall level of CD44 expression on the cell surface, and resulted in the suppression of lung metastasis. Consistent with these results, a high expression level of ESRP1 in tumour specimens was associated with a poor prognosis in breast cancer patients. Metastasis allows cancer cells to avoid oxidative damage caused by excess ROS in the primary tumour [48] , with metastatic cancer cells often being required to adapt to the selective pressure of the tumour microenvironment [19] . Neutrophils were recently shown to accumulate in the lung before the arrival of metastatic cells as well as to inhibit lung metastasis of 4T1 cells through NADPH-dependent H 2 O 2 generation [21] . Neutralization of such oxidative stress at potential sites of metastasis may thus be required for cancer cells to establish metastatic lesions. The cystine transporter xCT promotes GSH synthesis and ROS defence in cancer cells and thereby has a key role in resistance to cancer therapy [18] , [27] , and it has recently been implicated in cancer metastasis [49] . We found that ESRP1-dependent alternative splicing of CD44 mRNA increases both the intracellular GSH level and lung metastatic potential in breast cancer cells. Furthermore, forced expression of CD44v8-10 in ESRP1-depleted cells restored GSH content and lung metastatic ability to levels observed in ESRP1-replete cells. ESRP1-regulated alternative splicing of CD44 mRNA thus enhances xCT-dependent ROS defence and thereby allows cancer cells to evade metastatic stress. ALDH activity, in addition to CD44 expression, has been shown to be a marker for stem-like cells in breast cancer [38] . ALDH high CD44 + cells among human breast cancer cell lines show increased tumour formation and lung colonization abilities compared with ALDH low CD44 low/− cells [6] . We found that both CD44v + and CD44v − 4T1 cell subpopulations contain a small number of ALDEFLUOR-positive stem-like cells but that these stem-like cells among the CD44v + subpopulation underwent selective expansion in lung metastases. CD44v may therefore not be a specific marker for stem-like cancer cells but rather may be required to protect stem-like cells against oxidative stress. Induction of the EMT results in downregulation of ESRP1 expression [40] and thereby triggers a CD44 isoform switch from CD44v to CD44s in mammary epithelial cells [14] , [50] . Given that CD44v + and CD44v − 4T1 cells manifest similar expression levels of both epithelial and mesenchymal markers, the expression of ESRP1 as well as that of CD44v in these cells do not seem to be dependent on EMT status. ChIP sequencing analysis at the ESRP1 locus revealed that CD44v + cells manifest H3K4me3 (a mark of active transcription) at the transcription start site, whereas CD44v − cells manifest H3K27me3 (a mark of transcriptional repression). ESRP1 expression may thus be affected by the epigenetic status of the ESRP1 locus as well as by the EMT. Chromatin modifications including DNA and histone methylation at metastasis-related genes have been considered potential targets for the treatment of cancer metastasis [51] . Therapies targeted to the epigenetic regulation of ESRP1 as well as those that target CD44v-mediated stabilization of xCT might be expected to perturb the ROS resistance of metastatic stem-like cancer cells and thereby to render them susceptible to currently available cancer treatments. Cell culture The murine breast cancer cell line 4T1 (American Type Culture Collection, Rockville, MD) as well as CD44v + and CD44v − cells sorted therefrom were cultured under 5% CO 2 at 37 °C in RPMI 1640 medium (Sigma, St. Louis, MO) supplemented with 10% fetal bovine serum. 67NR, 168FARN, and 4T07 cells (kindly provided by Link Genomics, Tokyo, Japan) were cultured under 5% CO 2 at 37 °C in Dulbecco's modified Eagle's medium-F12 (Sigma) supplemented with 10% fetal bovine serum. Mice Wild-type Balb/c mice were obtained from CLEA Japan or Japan SLC (Tokyo, Japan). They were bred and maintained in the animal facility at Keio University according to institutional guidelines. All animal experiments were performed in accordance with protocols approved by the Ethics Committee of Keio University. Orthotopic transplantation and metastasis assay Parental, CD44v + , or CD44v − 4T1 cells (1×10 5 ) were orthotopically injected into the fourth mammary gland of syngeneic 8-to-10-week-old female wild-type Balb/c mice. At 30 days after transplantation, the mice were killed and the lungs removed. Quantification of lung metastasis was performed by imaging as described below. IntegriSense imaging Twenty-four hours before imaging, mice were injected intravenously with 2 nmol of IntegriSense 750 (VisEn Medical, Bedford, MA). Fluorescence imaging was performed with a ClairvivoOPT in vivo fluorescence imager (Shimadzu), with excitation at 785 nm with a laser diode and detection of fluorescence with an 845/55-nm band-pass filter. For quantitative comparisons, the total fluorescence signal intensity (pixel count) in a region of interest corresponding to each lung metastasis was measured. Tumour cell isolation and flow cytometry 4T1PT or 4T1LM cells were isolated from primary tumours or lung metastases, respectively, formed 30 days after orthotopic injection of 4T1 cells (1×10 5 ) into the mammary gland of recipient mice. Primary tumours or lung metastases were digested for 4 to 5 h at 37 °C in Ham's F12 medium supplemented with 5% fetal bovine serum, penicillin (100 U ml −1 ), streptomycin (100 μg ml −1 ), bovine insulin (5 μg ml −1 ), collagenase (300 U ml −1 ), and hyaluronidase (100 U ml −1 ). Red blood cells were then lysed by the addition of NH 4 Cl to a final concentration of 100 mM at room temperature, and tissue fragments were dissociated by gentle pipetting first in the presence of 0.25% trypsin for 1 to 2 min and then in the additional presence of dispase (5 mg ml −1 ) and DNase I (0.1 mg ml −1 ) for 2 min. All reagents were obtained from Stemcell Technologies (Vancouver, Canada). The mixture was then filtered through a 40-μm nylon mesh to yield a single-cell suspension, and the cells were cultured in the presence of 0.4 μM 6-TG (Sigma) for 2 to 3 days and then subjected to FACS to isolate Lin − cells. Cultured cells were dissociated by exposure to enzyme-free, Hanks-based Cell Dissociation Buffer (GIBCO-Invitrogen, Tokyo, Japan). For flow cytometric analysis or FACS, single-cell suspensions were incubated with antibodies for 20 min at 4 °C. Antibodies included phycoerythrin- and Cy7-conjugated antibodies to the lineage markers (Lin) CD31, CD45, and TER119 (BioLegend, San Diego, CA, USA), phycoerythrin-conjugated antibodies to pan-CD44 (IM7; eBioscience, San Diego, CA, USA), antibodies to xCT (Abcam, Cambridge, UK), allophycocyanin-conjugated antibodies specific for mouse CD44v [52] and fluorescein isothiocyanate-conjugated antibodies to human CD44v9 (ref. 18 ). Apoptotic cells were excluded for all flow cytometric analysis and FACS by elimination of cells positive for staining with propidium iodide. Flow cytometric analysis and FACS were performed with a FACSCalibur instrument (BD Biosciences, Tokyo, Japan) and either a FACSAria Cell Sorter (BD Biosciences) or MoFlo Cell Sorter (Beckman Coulter, Tokyo, Japan), respectively. For measurement of ROS or GSH levels, cells were incubated with 10 μM DCFH-DA or CFMDA (Invitrogen/Molecular Probes, Tokyo, Japan), respectively, for 15 min at 37 °C, washed twice with phosphate-buffered saline, and subjected to flow cytometric analysis. Immunoblot analysis Immunoblot analysis was performed, as described previously [53] , and with primary antibodies including those to pan-CD44 (IM7; BD Pharmingen, Tokyo, Japan; 500× dilution), E-cadherin (BD Pharmingen; 1,000× dilution), ZO-1, (Invitrogen, Tokyo, Japan; 1000× dilution), Twist (H-81; Santa Cruz Biotechnology, Santa Cruz, CA, USA; 200× dilution), N-cadherin (N-19; Santa Cruz; 1,000× dilution), Vimentin (BD Pharmingen; 200× dilution), and α-Tubulin (Sigma; 1,000× dilution). ALDEFLUOR assay An ALDEFLUOR kit (StemCell Technologies) was used to detect cells with a high ALDH activity. Cells were suspended in ALDEFLUOR assay buffer containing the ALDH substrate BODIPY aminoacetaldehyde (BAAA) and incubated for 40 min at 37 °C. As a negative control, cells were incubated in the additional presence of diethylaminobenzaldehyde (DEAB), a specific ALDH inhibitor. Imaging mass spectrometry 4T1 lung metastasis tissues snap-frozen in liquid nitrogen were dissected to prepare cryosections with 5-μm thickness by use of a cryostat (CM 1900; Leica Microsystems, Wetzlar, Germany). The sections were thaw-mounted on indium–tin oxide slides (Bruker Daltonik GmbH, Bremen, Germany) and were dried in silica gel-containing plastic tubes and, then, sprayed with 9-aminoacridine (9-AA, 20 mg in 4 ml 70% MeOH) by use of a 0.2-mm nozzle calibre airbrush (Procon boy FWA Platinum; Mr Hobby, Tokyo, Japan) to conduct matrix-assisted laser desorption/ionization (MALDI) imaging mass spectrometry in negative ion mode [34] , [35] . Adjacent sections were fixed with 4% buffered formalin (Nacalai Tesque, Kyoto, Japan) and stained with anti-CD44v antibody [52] . All the MALDI imaging experiments was carried out in negative-ion mode using a prototype Mass Microscope (Shimadzu Corporation, Kyoto, Japan). The laser power was adjusted to the desired intensities. MALDI mass spectra were acquired under the conditions laser diameter 10 μm, 80 shots per spot, scanning pitch 10 μm and scanning mass range from m / z 260 to m / z 670. Regions of the tissue samples exposed to the laser irradiation were determined by light microscopic observation. GSEA To detect overlap in gene expression profiles among multiple sets of genes, we used GSEA with the Kolmogorov-Smirnov enrichment algorithm and 400 random permutations to determine statistical significance. We first generated CD44v + /CD44v − log 2 ratio data from our microarray experiment and divided genes into those whose expression was upregulated (log 2 ratio >0) or downregulated (log 2 ratio <0). Second, we collected public microarray data (GSE11274 and GSE16925) from the GEO database and calculated the P -value ( t test) and log 2 ratio for ES cells/MEFs or iPS cells/MEFs with the use of the SAM R-package. We extracted the genes with a >2.0-fold change in expression (upregulated) or <0.5-fold change (downregulated) on average and a SAM P -value of <0.05. Third, up- or down-regulated gene sets in our CD44v + /CD44v − microarray experiment were compared with the ES and iPS cell signature gene sets by GSEA. ChIP sequencing and data analysis ChIP was performed as previously described [54] . CD44v + or CD44v − 4T1 cells were fixed with 1% formaldehyde, neutralized with 0.2 M glycine, and suspended in a lysis buffer containing 10 mM Tris–HCl (pH 8.0), 150 mM NaCl, 1% SDS, 1 mM EDTA, and a protease inhibitor cocktail (Roche, Tokyo, Japan). The cell lysates were subjected to ultrasonic treatment (Sonifier 250; Branson, Kanagawa, Japan) and diluted with a solution containing 20 mM Tris–HCl (pH 8.0), 150 mM NaCl, 1 mM EDTA, and 1% Triton X-100) for immunoprecipitation with Protein A/G (Invitrogen)-bound antibodies to H3K4me3 or to RNA polymerase II (both kindly provided by H. Kimura) or with those to H3K27me3 (Merck, Tokyo, Japan). Precipitated DNA was prepared according to the Illumina/Solexa Genomic DNA protocol (Illumina, San Diego, CA). The DNA was amplified by PCR (18 cycles) with annealing to the flow cell of a Genome Analyzer. DNA fragments of 350 to 450 bp were purified after separation on an agarose gel and diluted to 10 nM for loading on the flow cell. The DNA library (2 pM) was applied to the flow cell with the use of the Cluster Station device (Illumina). ChIP sequencing (ChIP-seq) data were analysed, as described [54] . In brief, images acquired from the Illumina/Solexa sequencer were processed through the bundled Solexa image extraction pipeline, which identified Polony positions, performed base-calling, and generated quality control (QC) statistics. Sequences were aligned with the human genome in the NCBI genomic database (UCSC mm9) as the reference genome. Sequences that mapped uniquely to the genome with two-base mismatches were selected. Sequences from all lanes for each ChIP sample were combined, extended 200 bp (maximum fragment length accounting for ~100 bp of primer sequence), and allocated into 25-bp bins. Genomic bins showing statistically significant ChIP-seq enrichment were identified by comparison with a Poissonian background model. For every 500-bp (for H3K4me3 and RNA polymerase II) or 1,000-bp (for H3K27me3) window, the mapped tag count for the ChIP sample ( C c ) and that for the ChIP input ( C i ) were used for calculation. E c and E i represent the estimated counts for 500-bp windows for the ChIP sample and ChIP input, respectively. The signal ratio was calculated as ( C c / E c +1)/Max(1, C i / E i +1). These signals were visualized with Integrated Genome Browser software (Affymetrix, Santa Clara, CA, USA) [55] . Statistical analysis Data are presented as means±s.d. and were analysed with the unpaired Student's t test. A P -value of <0.05 was considered statistically significant. Accession codes: The microarray data have been deposited in the GEO database under the accession code GSE35803 . How to cite this article: Yae, T. et al . Alternative splicing of CD44 mRNA by ESRP1 enhances lung colonization of metastatic cancer cell. Nat. Commun. 3:883 doi: 10.1038/ncomms1892 (2012).